Umpolung reactivity of strained C–C σ-bonds without transition-metal catalysis 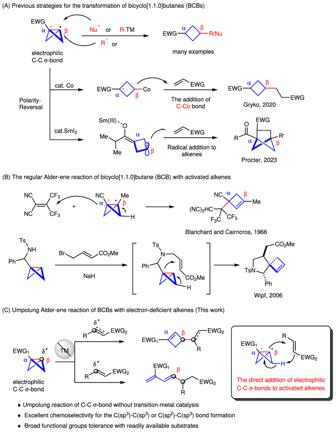Fig. 1: Transformation of strained C–C σ-bonds in BCBs. APrevious strategies for the transformation of bicyclo[1.1.0]butane (BCBs).BThe regular Alder-ene reaction of bicyclo[1.1.0]butanes (BCBs) with activated alkenes.CUmpolung Alder-ene reaction of BCBs with electron-deficient alkenes. Umpolung is an old and important concept in organic chemistry, which significantly expands the chemical space and provides unique structures. While, previous research focused on carbonyls or imine derivatives, the umpolung reactivity of polarized C–C σ-bonds still needs to explore. Herein, we report an umpolung reaction of bicyclo[1.1.0]butanes (BCBs) with electron-deficient alkenes to construct the C(sp 3 )-C(sp 3 ) bond at the electrophilic position of C–C σ-bonds in BCBs without any transition-metal catalysis. Specifically, this transformation relies on the strain-release driven bridging σ-bonds in bicyclo[1.1.0]butanes (BCBs), which are emerged as ene components, providing an efficient and straightforward synthesis route of various functionalized cyclobutenes and conjugated dienes, respectively. The synthetic utilities of this protocol are performed by several transformations. Preliminary mechanistic studies including density functional theory (DFT) calculation support the concerted Alder-ene type process of C–C σ-bond cleavage with hydrogen transfer. This work extends the umpolung reaction to C–C σ-bonds and provides high-value structural motifs. Umpolung reactions create new chemical space by reversing of the inherent polarity of a functional group [1] , [2] , [3] . This concept provides a different approach to access target products that would be difficult to obtain by classical processes. Previous reports have mainly focused on carbonyl groups [4] , [5] , imines [6] , [7] or amides [8] , other reactions especially to realize the polarized C–C σ-bond umpolung, have rarely been developed and would be of much more interest. Strain-release-driven reactions including cyclobutane, azetidine and bicyclo[1.1.1]pentane moieties have emerged as economical and efficient strategies for the construction of high-value molecular scaffolds, which are present in numerous natural products and pharmaceuticals [9] , [10] , [11] , [12] , [13] , [14] , [15] , [16] , [17] . Since Baran’s fundamental C–N bond formation through strain-release of the bridging C–C σ-bonds in bicyclo[1.1.0]butane (BCB) derivatives [18] , [19] , BCBs have gained significant attention from the synthetic community. BCBs have been used as privileged motifs to give functionalized cyclobutanes through nucleophilic addition [20] , [21] , [22] , [23] , [24] , [25] , radical addition [26] , [27] , [28] , [29] , [30] , coupling reactions with transition-metal catalysis [31] , [32] , [33] , [34] and others [35] , [36] , [37] , [38] , [39] . BCBs served as electrophiles or radical acceptors due to their inherent electrophilic reactivity, and all these reactions occur at the β-position of the bridging C–C σ-bonds. The polarity-reversal strategy for BCBs would offer new chemical space, but remains scarce (Fig. 1A ) [40] , [41] . In 2020, Gryko group developed the first polarity-reversal strategy of bicyclo[1.1.0]butanes (BCBs) by light-driven cobalt catalysis [40] . The in situ generation of the C–Co(III) bond is crucial for the polarity-reversal radical additions, but only gave poor diastereoselectivity of 1, 3-disubstituted cyclobutanes. Very recently, Procter group developed the SmI 2 –catalyzed radical addition of BCB ketones to electron-deficient alkenes to afford the substituted bicyclo[2.1.1]hexanes (BCHs), which are difficult to access by other approaches (Fig. 1A ) [41] . Fig. 1: Transformation of strained C–C σ-bonds in BCBs. A Previous strategies for the transformation of bicyclo[1.1.0]butane (BCBs). B The regular Alder-ene reaction of bicyclo[1.1.0]butanes (BCBs) with activated alkenes. C Umpolung Alder-ene reaction of BCBs with electron-deficient alkenes. Full size image Inspired by the previous rare examples of the direct regular addition of polarized C–C σ-bonds in bicyclo[1.1.0]butane (BCBs) to activated alkenes [42] , [43] , [44] , [45] , [46] , [47] , [48] , [49] , such as the intermolecular addition to 1,1-bis(trifluoromethyl)−2, 2-dicyanoethylene by Blanchard and Cairncross [43] , [44] and the intramolecular Alder-ene reaction to give spirocyclic compounds by Wipf (Fig. 1B ) [48] , [49] , we questioned whether the strain-release-driven strategy could enable umpolung reaction of the polarized C–C σ-bond with alkene. Herein, we report the umpolung reaction of BCBs with electron-deficient alkenes via Alder-ene process, delivering an array of two types of products: C(sp 3 )–C(sp 3 ) bond formation products (cyclobutenes) or C(sp 2 )–C(sp 3 ) bond formation products (conjugated dienes) (Fig. 1C ). Based on current mechanistic studies, we propose the reaction proceeds through the concerted cleavage of C–C σ-bonds with hydrogen transfer to deliver the cyclobutene products. Moreover, the conjugated dienes could also be obtained in one pot with just modified reaction conditions. Reaction investigations We initiated our studies by using bicyclo[1.1.0]butane (BCB) 1a as model substrate for the directed addition of C–C σ-bond to activated alkene 2a (Fig. 2 , for details see the Supplementary Table S1 ). After systematic investigations of the reaction parameters, we found that the polarity-reversal conjugate addition product 3a could be obtained in 91% yield with excellent regioselectivity when dimethyl sulfoxide (DMSO) was used as the solvent at 80 °C (entry 1). Control experiments showed that the addition of Na 2 SO 4 , MgSO 4 and 4 Å molecular sieves could decrease the decomposition of 1a and be benefit for the formation of 3a (entries 2–4). Other solvents did not give a better result than DMSO (entries 5–10). The yield of 3a was only 22% when the temperature was decreased to 50 °C, combined with starting materials recovered. The product 3a was obtained in very low yield when the reaction was performed at 100 °C, probably due to the decomposition of 1a at this temperature (entries 11 and 12). The concentration of this reaction was also important for efficiency (entry 13), and one equivalent of 1a only yielded 3a in 34% yield (entry 14). The yield of 3a could be increased to 66% with 4.0 eq of 2a (entry 15). 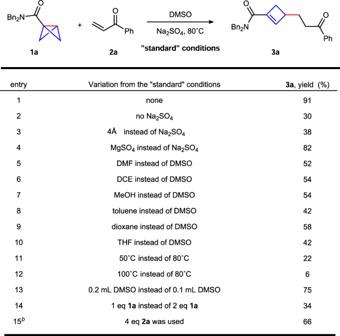Fig. 2: Optimization of reaction conditions.a aReaction conditions A: BCB1a(0.2 mmol), alkene2a(0.1 mmol), Na2SO4(0.17 mmol), 80 °C in DMSO (0.1 mL) under argon, 24 h, isolated yield.bReaction conditions B: BCB1a(0.1 mmol), alkene2a(0.4 mmol). Further increasing the equivalent of 2a did not improve the yield of 3a (for more details see the Supplementary Table S1 ). Fig. 2: Optimization of reaction conditions. a a Reaction conditions A: BCB 1a (0.2 mmol), alkene 2a (0.1 mmol), Na 2 SO 4 (0.17 mmol), 80 °C in DMSO (0.1 mL) under argon, 24 h, isolated yield. b Reaction conditions B: BCB 1a (0.1 mmol), alkene 2a (0.4 mmol). Full size image Substrates scope studies With the optimized reaction conditions in hand, we then explored the generality of this umpolung reaction (Fig. 3 ). Using bicyclo[1.1.0]butane 1a as a standard substrate, the scope of electro-deficient alkenes was examined and found to be very broad. A series of functional groups at the para -position of benzene rings worked well to give the desired products ( 3a – 3f , 51–91% yield). The meta - and ortho -substituted enones are also tolerated ( 3g – 3k , 44–68% yield). Hetero-aryl substituted enones also gave the corresponding products 3l – 3o in 58–85% yield. The alkenes with alkyl-substituted, ester or aldehyde group also worked smoothly to give C(sp 3 )–C(sp 3 ) bond formation products ( 3p – 3r , 39–72% yield). Other amide substituted BCBs were also investigated and found to be compatible with Weinreb amide ( 3s , 79% yield) and morpholine amide ( 3t , 70% yield). Besides amides, various electron-withdrawing groups such as sulfone, ester and nitrile were successfully converted to the corresponding products just with neat reaction conditions ( 3u , 12% yield; 3v , 42% yield and 3w , 24% yield). Aryl ketones and alkyl ketone attached BCBs also worked smoothly to give umpolung Alder-ene products ( 3x , 34% yield; 3xa , 59% yield; 3xb , 39% yield and 3xc , 34% yield) (for details see the Supplementary Tables S2 and S3 ). Given the long synthesis route of bicyclo[1.1.0]butanes, excess alkenes were used for several substrates (Reaction conditions B), but led to lower yield of desired products ( 3a , 66% yield; 3c , 41% yield; 3i , 39% yield; 3j , 65% yield; 3m , 60% yield; 3q , 19% yield and 3s , 67% yield). Noteworthy, the substituted alkyne is also suitable to be an acceptor in this reaction system and a high yield was obtained with excess of alkyne ( 3y , 72% yield). However, the reaction with electron-rich alkenes such as styrene and 1,1-diphenylethylene failed to give addition products, only with starting materials recovered. Fig. 3: Substrate scope of monosubstituted alkenes. a a Reaction conditions A: BCB 1 (0.2 mmol), alkene 2 (0.1 mmol), Na 2 SO 4 (0.17 mmol), 80 °C in DMSO (0.1 mL) under argon, 24 h, isolated yield. b 100 °C. c neat without any solvent, BCB 1 (0.1 mmol), alkene 2 (0.5 mmol), Na 2 SO 4 (0.17 mmol). d Reaction conditions B:BCB 1 (0.1 mmol), alkene 2 (0.4 mmol), Na 2 SO 4 (0.17 mmol), 80 °C in DMSO (0.1 mL). e MgSO 4 instead of Na 2 SO 4 . f 40 °C. Full size image To better define the application of this coupling system, we then examined the compatibility of more challenged 1, 2-disubstituted alkenes. The β-fluoroalkyl enones are attractive building blocks for the synthesis of high-value-added organofluorine compounds [50] , [51] , [52] , [53] . To our delight, these fluoroalkyl-containing enones are successfully applied in our systems, affording the C(sp 3 )–C(sp 3 ) bond formation products 4 and C(sp 2 )–C(sp 3 ) bond formation products 5 with excellent selectivity, respectively (Fig. 4 , for optimization of reaction conditions see the Supplementary Table S4 ). 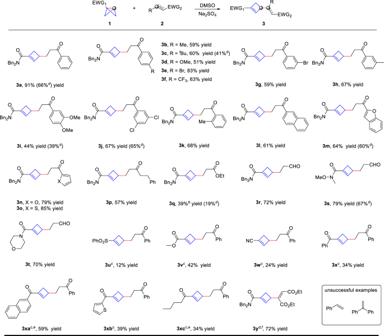Fig. 3: Substrate scope of monosubstituted alkenes.a aReaction conditions A: BCB1(0.2 mmol), alkene2(0.1 mmol), Na2SO4(0.17 mmol), 80 °C in DMSO (0.1 mL) under argon, 24 h, isolated yield.b100 °C.cneat without any solvent, BCB1(0.1 mmol), alkene2(0.5 mmol), Na2SO4(0.17 mmol).dReaction conditions B:BCB1(0.1 mmol), alkene2(0.4 mmol), Na2SO4(0.17 mmol), 80 °C in DMSO (0.1 mL).eMgSO4instead of Na2SO4.f40 °C. We first briefly examined the substrate scope to deliver cyclobutenes 4 . A series of enones bearing fluoro -, chloro -, electron-withdrawing and -donating groups at the para -position of the benzene ring worked smoothly to give formal 1, 4-conjugate addition products with excellent yield, moderate diastereoselectivity and excellent regioselectivity ( 4a – 4f , 74–99% yield, dr 5: 1, 4 : 5 = 8:1 to >20:1). The reaction also tolerated with 2-naphthyl-substituted enone ( 4g , 99% yield, dr 5: 1, 4 : 5 > 20:1). When the trifluoromethyl group was replaced by a pentafluoroethyl group, the desired cyclobutene 4 h was obtained in 98% yield and excellent diastereoselectivity ( dr 10:1, 4 : 5 > 20:1). Other electron-withdrawing groups such as Weinreb amide ( 4i , 36% yield), ester ( 4j , 21% yield) and alkyl ketone ( 4k , 34% yield) did lead to umpolung addition product formation, albeit with low yields. Interestingly, we got the C(sp 2 )–C(sp 3 ) bond formation diene product 5 when the reaction proceeded at higher temperature, and no cyclobutenes 4 were observed under this condition. Again, the substrate scope to access 5 was also found to be very broad. Various enones bearing halo- , electron-withdrawing and -donating groups were well tolerated ( 5a – 5h , 62–95% yield). The structure of 5g was unambiguously confirmed by X-ray crystallography (CCDC 2216789). The enones bearing fluoro- , chloro- , and trifluoromethyl groups at the meta- position of the benzene rings gave the desired products in moderate yield ( 5i – 5k , 67–68% yield). The introduction of a substituent at the ortho position resulted in slightly diminished yield ( 5l – 5n , 47–69% yield), likely due to the steric hindrance effect. The 2-naphthyl- and furyl-substituted enones afforded the corresponding products in acceptable yield ( 5o , 54% yield and 5p , 44% yield). An array of functionalized β-pentafluoroethyl enones also successfully led to the diene products ( 5q – 5u , 44–64% yield). However, the less reactive ( E )−1-phenylbut-2-en-1-one, chalcone and bicyclo[2.1.0]pentane all failed to give conjugate addition products and dienes. 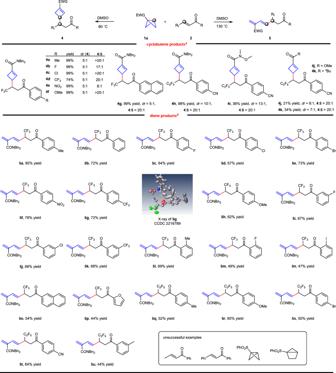Fig. 4: Substrate Scope of 1, 2-disubstituted alkenes.a aReaction conditions: BCB1(0.3 mmol), alkene2(0.1 mmol), Na2SO4(0.17 mmol), 80 °C in DMSO (0.1 mL) under argon, 48 h, isolated yield.bReaction conditions: BCB1(0.2 mmol), alkene2(0.1 mmol), Na2SO4(0.17 mmol), 130 °C in DMSO (1.0 mL) under argon, 48 h, isolated yield. These results in the Synthetic applications and Computational studies indicated diene product 5a was formed from 4a through electrocyclic ring-opening process. Fig. 4: Substrate Scope of 1, 2-disubstituted alkenes. a a Reaction conditions: BCB 1 (0.3 mmol), alkene 2 (0.1 mmol), Na 2 SO 4 (0.17 mmol), 80 °C in DMSO (0.1 mL) under argon, 48 h, isolated yield. 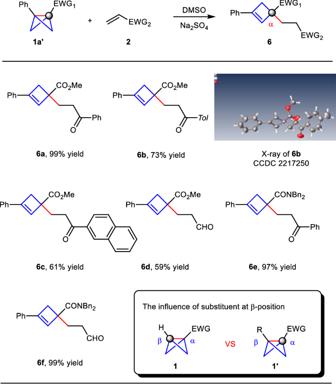Fig. 5: The influence of the substituent at the β-position of bicyclo[1.1.0]butanes.a aReaction conditions: BCB1a’(0.2 mmol), alkene2(0.1 mmol), Na2SO4(0.17 mmol), 80 °C in DMSO (0.1 mL) under argon, 24 h, isolated yield. b Reaction conditions: BCB 1 (0.2 mmol), alkene 2 (0.1 mmol), Na 2 SO 4 (0.17 mmol), 130 °C in DMSO (1.0 mL) under argon, 48 h, isolated yield. Full size image Furthermore, we investigated the influence of the substituent at the β-position of BCBs in this umpolung reaction. As shown in Fig. 5 , with the 1,3-disubstituted bicyclobutane 1a’ , some differently substituted enones and acrolein worked well to deliver the regular addition products at the α-position of the electron-withdrawing group ( 6a–6d , 59–99% yield), but not the polarity-reversal addition products at the β-position [54] , [55] , [56] , [57] . The structure of 6b was confirmed by X-ray crystallography (CCDC 2217250). Moreover, the amide group attached to BCBs proved to be viable substrates, providing addition products in excellent yield ( 6e , 97% yield and 6f , 99% yield). These results indicated the steric hindrance of the substituent at the β-position would change the regioselectivity of the bridging C–C σ-bond in our reaction systems. Fig. 5: The influence of the substituent at the β-position of bicyclo[1.1.0]butanes. a a Reaction conditions: BCB 1a’ (0.2 mmol), alkene 2 (0.1 mmol), Na 2 SO 4 (0.17 mmol), 80 °C in DMSO (0.1 mL) under argon, 24 h, isolated yield. Full size image Synthetic applications This polarity-reversal C–C σ-bond involved in the conjugate addition reaction turned out to be synthetically useful (Fig. 6 ). The reaction was readily scaled up to 6.0 mmol, giving the cyclobutene product 3r in 70% yield and the diene product 5a in 76% yield, respectively. The diene product 5a could be obtained quantitatively from 4a through an electrocyclic ring-opening process and was ready to undergo isomerization under base conditions to give product 7 in 42% yield. The cyclobutene 3r was successfully hydrogenated by H 2 to give cyclobutane product 8 in 73% yield and 10:1 dr in the presence of Pd/C catalyst. When Raney-Ni was used, the reduction of carbonyl group and double bond occurred in one pot to give cyclobutane product 9 in 68% yield and 17:1 dr [58] , [59] . Other reactions such as Wittig-reactions were also successfully performed, giving the product 10 in 93% yield or terminal alkene 11 in 81% yield. The selective reduction of carbonyl group with NaBH 4 could give the alcohol product 12 in 85% yield, which would undergo cyclization under base conditions to access bicyclic product 13 in 90% yield and 6:1 dr . Fig. 6: Synthetic applications. Scale-up synthesis and derivatization of 3r . Full size image Mechanistic studies Then we conducted several experiments to probe the reaction mechanism [38] , [39] , [40] , [41] . When CF 3 CD 2 OD was used as solvent or 20.0 eq CD 3 CO 2 D was added in DMSO solvent, no deuterium incorporation was detected in the product 3a , which excludes the carbanion species in the reaction (Fig. 7A ). Besides, several radical-probe experiments were performed. The reaction of 1a and 2a was found to be essentially unaffected by the addition of 1, 1-diphenylethylene, BHT or TEMPO (2, 2, 6, 6-tetramethyl-1-piperidinyloxy) (Fig. 7B ). The cyclopropyl-containing alkene 2y was also successfully applied to deliver the 1, 4-conjugate addition products 14 and 15 without the cleavage of C–C bond in cyclopropyl group. Furthermore, the phenyl-substituted 2y’ was further used to probe the radical pathway, which also delivered cyclopropyl-containing products 16 and 17 (Fig. 7C ). EPR experiments showed no radical signal observed for the formation of products 3a, 6a, 16 and 17 (for more details see Supplementary Figs. 41 – 44 ) (Fig. 7D ) [60] . In addition, kinetic studies of the reaction of BCB 1a and enone 2aa exhibited first-order kinetics for both BCB 1a and 2aa , indicating that both BCB and alkene are involved in the turnover-limiting step (Fig. 7E ). These kinetic results are consistent with the density functional theory (DFT) calculations results in Fig. 8 . The experimentally measured activation free energy from the Eyring equation ( ΔG exp ‡ = 28.1 kcal/mol, for more details see the Supplementary Figs. 45 – 49 ), these results agree with the DFT calculation of the energy barrier ( TS1 in Fig. 8 , ΔG ‡ = 27.9 kcal/mol) (Fig. 7F ) [61] . Fig. 7: Mechanistic studies. A Deuterium experiments. B Radical-probe experiments. C Radical clock experiments. D EPR experiments. E Kinetic studies. F The experimentally measured Gibbs free energy. 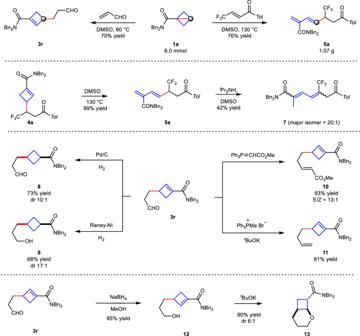Fig. 6: Synthetic applications. Scale-up synthesis and derivatization of3r. Full size image Fig. 8: Computational studies. The corresponding energy profiles of the chemoselective pathways for the selected model reaction between BCB 1a and β-trifluoromethyl enone 2aa . Full size image Theoretical calculations were performed to investigate the detailed mechanism of this umpolung addition (for more computational details, see the Supporting Information). As shown in Fig. 8 , both the α site and β site of 1a were considered to undergo an Alder-ene type reaction with alkene 2aa , where the middle C–C σ bond cleavage in BCB 1a was broken accompanying by a hydrogen transfer from four-membered ring to alkene. The computational results demonstrate that the energy barrier of Alder-ene type reaction on β site via transition state TS1 ( ΔG ‡ = 27.9 kcal/mol) is 6.9 kcal/mol lower than that on α site via transition state TS1′ ( ΔG ‡ = 34.8 kcal/mol). Therefore, 4a is the main product in kinetically, which is consistent with the chemoselectivity in experiment. In addition, when the reaction temperature is raised from 80 °C to 130 °C, the four-membered ring opening of 4a could irreversibly occur to generate the diene product INT1 via pericyclic transition state TS2 ( ΔG ‡ = 32.9 kcal/mol). Isomerization of diene INT1 would give the diene product 5a . All the calculated results are consistent with the experimental results. When the BCB substrate has a phenyl group at the β site ( 1a’ ), the Alder-ene type reaction at the α site should be more energetically favorable to deliver the product 6a , and the regioselectivity could be reversed by replacing the substrate 1a with 1a′ having a phenyl substituent at the β site, probably due to the steric hindrance effect, which is also in agreement with the experimental result (for more details see the Supplementary Fig. 57 ). During our submission, Anderson’s group also discovered the stereoselective Alder-ene reactions of bicyclo[1.1.0]butanes with strained alkenes and alkynes. The regioselectivity is the same as our product 6 in Fig. 5 and their mechanism studies also support an Alder-ene process, not a radical pathway [62] . The concerted transition state of the C–C σ bond cleavage in BCBs together with hydrogen transfer contributes to the chemoselectivity. In summary, we have developed a formal 1,4-conjugate addition of polarity-reversal C–C σ-bond to activated alkene under very simple reaction conditions without transition-metal catalysis, in which the strain-release-driven strategy is crucial for this neutral transformation. The umpolung reaction of C–C σ-bonds in bicyclo[1.1.0]butanes (BCBs) with various electrophilic alkenes, provides an atom-economic and straightforward approach for the synthesis of cyclobutenes and conjugated dienes with excellent selectivity. Mechanistic studies showed that a concerted Alder-ene type process would be the most likely pathway to give these formal conjugate addition products. We anticipate that this synthetic protocol will enhance chemists’ tools for classic umpolung reactions. From a broader perspective, we envision that this umpolung reaction of strained C–C σ-bonds strategy will prove applicable in both modern synthetic chemistry and pharmaceutical research. Umpolung reactions of polarized C–C σ-bonds with activated alkenes 1a (0.2 mmol), 2 (0.1 mmol), Na 2 SO 4 (0.17 mmol) in DMSO (0.1 mL) were charged into a pressure tube under argon. The reaction tube was then sealed and placed into an oil bath at 80 °C. After being stirred for 24 h, the reaction vessel was removed from the oil bath and cooled to ambient temperature. To the reaction mixture, H 2 O (4.0 mL) was added, and the mixture was extracted with Et 2 O. The organic layer was concentrated and purified by silica gel chromatography (PE: EA = 5:1) to give the indicated product 3 or 6 . More details and characterization of the products are available in the Supplementary Information. 1a (0.3 mmol), 2 (0.1 mmol), Na 2 SO 4 (0.17 mmol) in DMSO (0.1 mL) were charged into a pressure tube under argon. The reaction tube was then sealed and placed into an oil bath at 80 °C. After being stirred for 24 h, the reaction vessel was removed from the oil bath and cooled to ambient temperature. To the reaction mixture, H 2 O (4.0 mL) was added, and the mixture was extracted with Et 2 O. The organic layer was concentrated and purified by silica gel chromatography (PE: EA = 5:1) to give the indicated product 4 , More details and characterization of the products are available in the Supplementary Information. 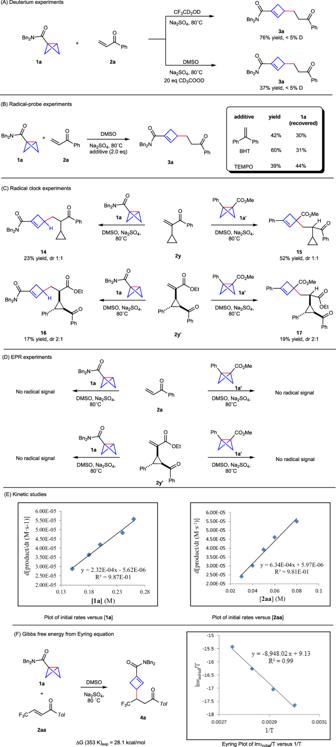Fig. 7: Mechanistic studies. ADeuterium experiments.BRadical-probe experiments.CRadical clock experiments.DEPR experiments.EKinetic studies.FThe experimentally measured Gibbs free energy. 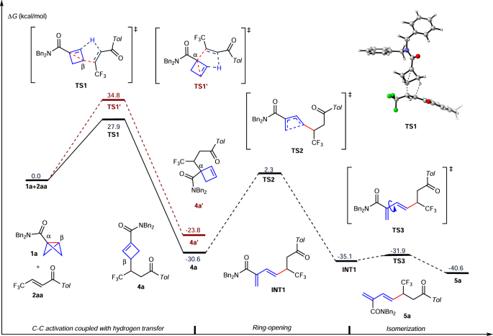Fig. 8: Computational studies. The corresponding energy profiles of the chemoselective pathways for the selected model reaction between BCB1aand β-trifluoromethyl enone2aa. 1a (0.2 mmol), 2 (0.1 mmol), Na 2 SO 4 (0.17 mmol) in DMSO (1.0 mL) were charged into a pressure tube under argon. The reaction tube was then sealed and placed into an oil bath at 130 °C. After being stirred for 48 h, the reaction vessel was removed from the oil bath and cooled to ambient temperature. To the reaction mixture, H 2 O (4.0 mL) was added, and the mixture was extracted with Et 2 O. The organic layer was concentrated and purified by silica gel chromatography (PE: EA = 5:1) to give the indicated product 5 . More details and characterization of the products are available in Supplementary Information.